Direct contribution of the seagrassThalassia testudinumto lime mud production Seagrass beds contribute to oceanic carbonate lime mud production by providing a habitat for a wide variety of calcifying organisms and acting as efficient sediment traps. Here we provide evidence for the direct implication of Thalassia testudinum in the precipitation of aragonite needles. The crystals are located internally in the cell walls, and as external deposits on the blade, and are similar in size and shape to the aragonite needles reported for modern tropical carbonate factories. Seagrass calcification is a biological, light-enhanced process controlled by the leaf, and estimates of seagrass annual carbonate production in a Caribbean reef lagoon are as significant as values reported for Halimeda incrassata . Thus, we conclude that seagrass calcification is another biological source for the aragonite lime mud deposits found in tropical banks, and that tropical seagrass habitats may play a more important role in the oceanic carbon cycle than previously considered. As a substantial component of carbonate sediments throughout the geological record [1] , lime mud plays a significant role in the capacity of the ocean to store and cycle carbon. Several processes are directly involved in the diverse origin of lime mud, including physico-chemical precipitation [2] , [3] , bacterial–microalgal activity [4] , breakdown of large skeletal bioclasts (for example, foraminifera) [1] , disintegration of thinly calcified skeletons [5] , [6] , [7] , [8] and/or the decomposition of fish pellets [9] . A recent global characterization of modern carbonate mud deposits from reefs and carbonate platforms concluded that modern tropical muds are largely derived from the breakdown of skeletal grains and the disintegration of codiacean algae [10] . This conclusion was based on the composition of the finest fraction (<4 μm), which was predominated by aragonite needles, nanograins and coccoliths [10] . Only carbonate mud from the Great Barrier Reef (GBR) and Northern Belize differed from other mud deposits in terms of elevated amounts of high-magnesium calcite and lower aragonite, strontium and δ 13 C values [10] , although in Northern Belize the finest fraction was absent. In contrast, Bahamian sediments showed the highest aragonite (95.3%) and strontium (6,000 p.p.m.) content [10] . The current hypothesis regarding the Florida-Bahamas system is that spontaneous chemical precipitation is the primary origin of the lime mud sediments [3] , [10] . However, strontium content and δ 13 C in the Bahamas are below the expected values for non-skeletal grains (that is, 6,000<9,000 p.p.m. and +2‰<+5‰, respectively) [10] . This finding indicates that a biological skeletal source must also be involved in the origin of these sediments. Seagrass habitats contribute significantly to the formation of lime mud [11] , [12] through the provision of a habitat for diverse and productive calcifying organisms [11] , [13] , [14] , the promotion of sedimentation by reducing water flow [13] , [15] and the stabilization of sediments by roots and rhizomes. However, the large volume of the Holocene aragonitic-mud deposits accumulated on the Great Bahama Bank (GBB) [16] cannot be explained by the productivity of the seagrass-calcifying algae and/or infauna alone. The current standing biomass of Penicillus capitatus and Halimeda incrassata , common in seagrass beds dominated by the turtlegrass Thalassia testudinum, is too low to account for the carbonate accumulation in the Holocene lime mud bank [17] , [18] . These codiacean algae were initially proposed as the major source of the Bahamian carbonate sediments [5] , [6] , [7] , [8] , but further comparison of algae and mud deposits reported large differences between the algal needles and the sedimentary crystals in terms of morphology [18] , [19] , biochemistry [20] and isotopic fractionation [18] . An alternative biological source for the sediments is the epibiont community [11] , [12] , [14] developed on the seagrass blades. Epibiont carbonate production can be equal to or greater than estimates for codiacean algae [9] , [14] , [21] . However, the dominant calcifying epibionts on T. testudinum leaves are encrusting Mg-calcite red algae with minor contributions from aragonitic bryozoans and serpulids, limiting the capacity of the seagrass epibionts to explain the Bahamian aragonite lime mud component of biological origin. Spontaneous chemical precipitation has also been considered as an important source of tropical lime mud sediments [3] . Supersaturated levels of calcium carbonate characterize the shallow, warm and hypersaline waters of modern carbonate factories, where events of drifting clouds of milky water created by the presence of suspended carbonate, called whitings, are frequent. Whitings are particularly common in the NW-W of Andros Island in Bahamas [18] , [22] and in Northern Belize [23] . Locally, they are known as fish-muds and explained by fishermen, as being sediment stirred-up by schools of bottom-feeding fishes. However, sediment re-suspension by fishes, wind, waves, tides and so on cannot explain their long persistence (>70 h) [18] . Estimations of carbonate precipitation from whitings in the Bahamas [22] are similar to the lime mud accumulation rates of the GBB [3] , [8] ; therefore, whitings are considered fundamental for the operation of the tropical carbonate factory [18] , [22] . A large body of evidence supports a sedimentary origin for whitings [7] , [18] , [19] , [20] . Radiocarbon dating has confirmed that the suspended carbonate is mainly derived from bottom sediments [7] ; however, active spontaneous CaCO 3 precipitation has been proposed as an alternative hypothesis to explain the presence of this suspended carbonate [18] , [22] . The CO 2 partial pressure within whitings does not differ from the surrounding water [7] , and oxygen-isotopic composition analyses have indicated that the suspended carbonate is not in equilibrium with the surrounding water [8] , [18] . Neither finding supports the active spontaneous precipitation hypothesis. Alternative hypotheses such as microbial lime-mud production [24] , wind-driven Langmuir cells [25] , and/or cyanobacteria blooms [26] , are not yet sufficiently tested. As the mechanism propelling the re-suspension and long persistence of the crystals in the water column [18] remains unknown, a controversial long-standing debate has been maintained in the literature regarding the origin of whitings and this suspended carbonate [7] , [12] , [18] , [26] , [27] . A similar long-standing debate still persists regarding the origin of the sedimentary crystals in modern tropical banks [6] , [7] , [8] , [18] , [28] . In this context, seagrass meadows seem to play a minor role in the operation of the tropical carbonate factory. Moreover, seagrasses seem to play a negative rather than positive role for the accumulation of carbonate lime mud, as a positive correlation between T. testudinum biomass and sediment carbonate dissolution has been documented [29] . This association is probably related to increases in organic matter oxidation, CO 2 release by the underground biomass, as well as the pH reduction observed in sediment-pore waters within turtlegrass beds [30] . Here we demonstrate the direct contribution of the tropical seagrass T. testudinum to lime mud production. We document for the first time that seagrass leaves are capable of inducing CaCO 3 precipitation in the form of small aragonite needles that match the shape and size of sedimentary crystals. Therefore, seagrass calcification should be considered another biological source for the aragonite lime mud deposits found in tropical banks. Estimates of annual carbonate production in a Caribbean reef lagoon from seasonal changes in seagrass calcification rates are similar to values reported for H. incrassata . These findings suggest that tropical seagrass habitats may play a more important role in the oceanic carbon cycle than previously thought. Seagrass calcification measurements and seasonal monitoring To reach these conclusions, we first measured leaf calcification rate using the alkalinity anomaly technique [31] . The first estimations determined in October 2008 for leaves collected in a coral reef lagoon (Puerto Morelos, Mexican Caribbean) showed an average value of 0.59±0.07 μmol CaCO 3 cm −2 h −1 . Using this methodology, we monitored seasonal variation in leaf calcification for a seagrass bed located in the back-reef of the lagoon (10 samplings from March to December 2009, and 9–10 determinations per sampling, Fig. 1 ). The estimated annual average rate for 2009 was 0.35±0.05 μmol CaCO 3 cm −2 h −1 , with a maximum rate of 0.48±0.08 μmol CaCO 3 cm −2 h −1 measured on June 2009. No significant differences were observed between this 2009 maximum and the value determined in October 2008 ( t -test, P >0.05, Fig. 1a,c ). This monitoring unveiled large seasonal variation in seagrass calcification: positive calcification was detected in May, June and August 2009; no significant changes in the alkalinity were observed in March and November 2009; and negative values were measured in July 2009 at high water temperature, and in the coldest months of March and December 2009 ( Fig. 1a ). Unfortunately, no data are available for September and October 2009, as no measurements were performed for these months. Temperature seems to enhance seagrass calcification but is not the main driver, as calcification was suppressed in summer (July) under high water temperature ( Fig. 1a ). A significant reduction in water motion was observed from April to September 2009 ( r =−0.45; P <0.01; Fig. 1b ) associated with the summer increment in the reef lagoon water temperature. However, water motion was not able to explain the negative values observed in July 2009 ( Fig. 1b ). Thus, no clear association was found between water temperature and/or water motion and seagrass calcification. The summer suppression in leaf calcification coincided with the highest gross photosynthesis determined in leaf incubations ( Fig. 1b ). 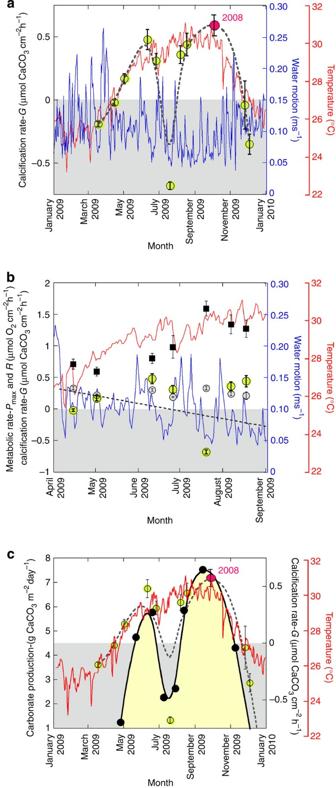Figure 1: Seasonal variation in seagrass calcification. Data shown are for leaves collected in 2009 in the back reef of the Puerto Morelos reef lagoon (Mexican Caribbean). Variation in water temperature (red line) and water motion (blue line) is also described for 2009. (a) Mean (±s.e.) variation of leaf calcification rates (n=9–10 leaf determinations per sampling) ofThalassia testudinumis represented with yellow circles. Dark pink circle represents the mean (±s.e.) for calcification rate ofT. testudinumperformed in October 2008. The grey shaded area indicates negative values for seagrass calcification, interpreted as decalcification. The dashed black line describe the annual pattern of variation in seagrass calcification. (b) Mean (±s.e.) of seagrass calcification rates (yellow cycles), gross photosynthesis (black squares) and leaf respiration (grey circles) determined between April 2009 to September 2009. The grey shaded area represents negative values for seagrass calcification. The dashed black line describes the linear fit for the variation in water motion. (c) Estimations of seagrass carbonate production (black circles) for 2009 for the seagrass meadow (number 5 inTable 1) located in the back reef of the lagoon. Values were calculated from the average of two consecutive determinations of leaf calcification rates (yellow circles) and the number of days elapsed between sampling periods. The October 2008 determination is also shown with a dark pink circle. The dashed black line represents the annual pattern of variation for seagrass calcification and the grey area identifies the negative values. Positive seasonal carbonate production is represented by the yellow shaded area. The solid black line describes the annual pattern of variation for gross carbonate production. Variation in water temperature (°C) and water motion (m s−1) was recorded by the Oceanographic and Meteorological Academic Service (SAMMO) of the UNAM Academic Unit in Puerto Morelos. Water temperature was recorded at 3.3 m depth in the middle of the reef lagoon, and water motion was registered with an Acoustic Doppler Velocimeter (Argonaut-ADV, SonTek/YSI). Measurements were made at 2 cm from the sediment, using a 6 mm diameter × 9 mm high cylinder. Figure 1: Seasonal variation in seagrass calcification. Data shown are for leaves collected in 2009 in the back reef of the Puerto Morelos reef lagoon (Mexican Caribbean). Variation in water temperature (red line) and water motion (blue line) is also described for 2009. ( a ) Mean (±s.e.) variation of leaf calcification rates ( n =9–10 leaf determinations per sampling) of Thalassia testudinum is represented with yellow circles. Dark pink circle represents the mean (±s.e.) for calcification rate of T. testudinum performed in October 2008. The grey shaded area indicates negative values for seagrass calcification, interpreted as decalcification. The dashed black line describe the annual pattern of variation in seagrass calcification. ( b ) Mean (±s.e.) of seagrass calcification rates (yellow cycles), gross photosynthesis (black squares) and leaf respiration (grey circles) determined between April 2009 to September 2009. The grey shaded area represents negative values for seagrass calcification. The dashed black line describes the linear fit for the variation in water motion. ( c ) Estimations of seagrass carbonate production (black circles) for 2009 for the seagrass meadow (number 5 in Table 1 ) located in the back reef of the lagoon. Values were calculated from the average of two consecutive determinations of leaf calcification rates (yellow circles) and the number of days elapsed between sampling periods. The October 2008 determination is also shown with a dark pink circle. The dashed black line represents the annual pattern of variation for seagrass calcification and the grey area identifies the negative values. Positive seasonal carbonate production is represented by the yellow shaded area. The solid black line describes the annual pattern of variation for gross carbonate production. Variation in water temperature (°C) and water motion (m s −1 ) was recorded by the Oceanographic and Meteorological Academic Service (SAMMO) of the UNAM Academic Unit in Puerto Morelos. Water temperature was recorded at 3.3 m depth in the middle of the reef lagoon, and water motion was registered with an Acoustic Doppler Velocimeter (Argonaut-ADV, SonTek/YSI). Measurements were made at 2 cm from the sediment, using a 6 mm diameter × 9 mm high cylinder. Full size image Seagrass calcification is considered a by-product of leaf photosynthesis [32] because of the CaCO 3 supersaturation associated with inorganic carbon uptake (that is, CO 2 uptake results in an increase in local pH, and HCO 3 − uptake is often coupled to OH − extrusion). In this scenario, seagrass calcification could be an artefact induced by leaf photosynthesis during incubation in small-volume chambers. However, we observed negative values, interpreted as decalcification, in the leaves collected in July 2009, showing the highest photosynthetic activity for leaves grown and incubated at high water temperature ( Fig. 1a ). If calcification was an artefact during incubation, samples from July 2009 would have shown the highest rates. Thus, it is possible that leaf calcification plays an unknown role in the photosynthetic metabolism of T. testudinum . While the biological mechanism between seagrass calcification and photosynthesis requires a physiological approach not conducted here, this relationship was analysed by measuring the instantaneous calcification rate under illumination, darkness and by using a known specific inhibitor of photosynthesis, the herbicide DCMU (see methods). We confirmed that under illumination, calcification increased to twice the basal rate observed under dark conditions ( Fig. 2a ). The suppression of photosynthesis with DCMU reduced the calcification rate to darkness levels (Student’s t -test, P >0.05, Fig. 2a ). Thus, we concluded that seagrass calcification is a light-enhanced process similar to what has been previously described for other marine calcifiers [33] , [34] , [35] . Seagrass photosynthesis enhances seagrass calcification but is not the main driver, as calcification also occurs in darkness and under photosynthesis suppression. To further understand the role of seagrass calcification in the photosynthetic metabolism of T. testudinum , we increased carbon limitation on seagrass photosynthesis by using an inhibitor of the external activity of the enzyme carbonic anhydrase, acetazolamide (AZ). Carbonic anhydrases (CA) are ubiquitous metalloenzymes that catalyse the reversible hydration of CO 2 into bicarbonate, and can act as a carbon concentration mechanism (CCM) for maintaining aquatic photosynthesis activity. External CA activity has been previously documented for T. testudinum leaves [36] . After acetazolamide (AZ) addition, we observed, as expected, a 35% reduction in leaf photosynthesis ( P max control=1.94±0.14 μmol O 2 cm −2 h −1 ; P max +AZ treated leaves=1.26±0.18 μmol O 2 cm −2 h −1 ). However, we also observed the complete inhibition of seagrass calcification, with large negative values attributed to decalcification ( Fig. 2a ). Previous studies have documented external CA activity in the calcification process mediated by the biology of an organism, from invertebrates to vertebrates [37] , suggesting that CA activity may play a key role in biomineralization. Our results support this interpretation, as this enzyme or a protein AZ-sensitive is also involved in seagrass calcification. We confirm that T. testudinum calcification is a biologically controlled process [38] , invalidating the assumption that it can be only explained as a by-product of seagrass photosynthesis or as an artefact of the leaf incubations. The genetic expression or suppression of a putative mechanism responsible for seagrass calcification could explain the seasonal variability found and also the negative values observed in the July 2009 leaves grown under high water temperature and that also showed high photosynthetic activity ( Fig. 1a ). 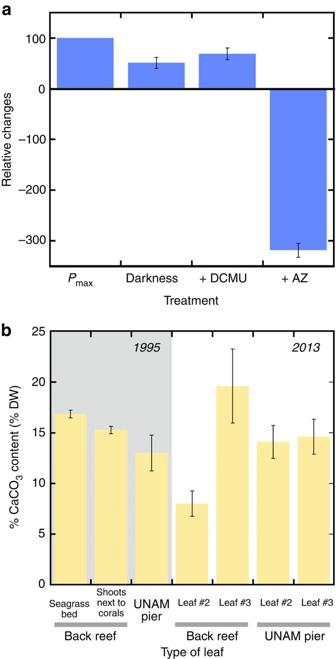Figure 2: Experimental responses and variation in leaf CaCO3content. (a) Relative changes (percentage) in the instantaneous calcification rates ofT. testudinumleaves with respect to the maximum calcification rate of the control leaf fragments, determined under maximum photosynthesis activity (Pmax). Leaf segments were incubated at 28 °C for 30 min under saturating irradiance (500 μmol quanta m−2s−1), and in darkness. Leaf segments were infiltrated for 10 min in darkness with the herbicide DCMU and treated with Acetazolamide (+AZ), an inhibitor of the extracellular activity of the enzyme carbonic anhydrase, before incubation under similar light conditions as the control. Each determination was replicated four times. (b) Mean±s.e. (n=9–12) of the percentage of leaf CaCO3content (% dry weight, DW) estimated for leaves of the seagrassThalassia testudinumcollected in the reef lagoon of Puerto Morelos (Mexican Caribbean) in May 1995 and in September 2013. Grey background shows values determined for the second youngest leaf collected in 1995, in the back reef, either in the seagrass bed or adjacent to massive coral colonies (shoots next to corals) and in a meadow adjacent to the UNAM pier. Comparisons between values of the CaCO3content variation between the second and third leaves of shoots collected in 2013 (#3 is the oldest leaf of the shoot) are also shown. Figure 2: Experimental responses and variation in leaf CaCO 3 content. ( a ) Relative changes (percentage) in the instantaneous calcification rates of T. testudinum leaves with respect to the maximum calcification rate of the control leaf fragments, determined under maximum photosynthesis activity ( P max ). Leaf segments were incubated at 28 °C for 30 min under saturating irradiance (500 μmol quanta m −2 s −1 ), and in darkness. Leaf segments were infiltrated for 10 min in darkness with the herbicide DCMU and treated with Acetazolamide (+AZ), an inhibitor of the extracellular activity of the enzyme carbonic anhydrase, before incubation under similar light conditions as the control. Each determination was replicated four times. ( b ) Mean±s.e. ( n =9–12) of the percentage of leaf CaCO 3 content (% dry weight, DW) estimated for leaves of the seagrass Thalassia testudinum collected in the reef lagoon of Puerto Morelos (Mexican Caribbean) in May 1995 and in September 2013. Grey background shows values determined for the second youngest leaf collected in 1995, in the back reef, either in the seagrass bed or adjacent to massive coral colonies ( shoots next to corals ) and in a meadow adjacent to the UNAM pier. Comparisons between values of the CaCO 3 content variation between the second and third leaves of shoots collected in 2013 (#3 is the oldest leaf of the shoot) are also shown. Full size image Estimations of seagrass carbonate budgets We calculated the daily and annual gross carbonate production for nine seagrass beds of the Puerto Morelos reef lagoon, using an estimated annual average value and integrating the carbonate production between two consecutive samplings ( Table 1 , see description in Methods). Selected seagrass meadows encompass the whole morphological variability displayed by the above-ground biomass of T. testudinum in this reef lagoon [39] . Differences observed in total leaf area (Leaf Area Index, LAI) were due to differential variation in shoot size and shoot density [39] . Values estimated for the back reef meadow are shown in Fig. 1c (number 5 in Table 1 ). This exercise revealed large seasonal and spatial variations in seagrass lime mud production, with values between 0.5 and 5.6 kg m −2 year −1 . This carbonate production is similar in magnitude to values reported for H. incrassata from this area (0.05–2.3 kg m −2 year −1 ) [40] , for coral reef environments (0.8–4 kg m −2 year −1 ) [41] , and is in the lower range of the values reported for scleractinian corals (5–30 kg m −2 year −1 ) [42] . Table 1 Variation in gross carbonate production for nine meadows located in a Caribbean reef lagoon. Full size table Loss on ignition analysis The absence of studies focusing on seagrass calcification can be attributed to the importance of seagrass epibionts for carbonate sediment production [11] , [14] , overshadowing the potential direct contribution of the seagrass leaf to those sediments. However, high leaf ash content is a general characteristic of aquatic leaves [43] and of tropical seagrasses in general [44] , [45] . T. testudinum has shown values often above 20% of the leaf dry weight [45] , [46] . The current study confirms that CaCO 3 content is a significant component of the T. testudinum leaf ash by measuring the differential loss of organic carbon and carbonate content through progressive sample ignition (loss on ignition technique, LOI [47] ). LOI analysis revealed significant differences among sites, shoot types and leaves in leaf CaCO 3 content ( Fig. 2b , analysis of variance (ANOVA), P <0.001). Leaf number 3 (#3) collected in September 2013 in the back reef of the Puerto Morelos reef lagoon showed the highest CaCO 3 content, significantly higher than leaf #2 from the same shoot. However, these high values were not significantly different from the leaf content determined in 1995 for leaf #2 from shoots collected in the back reef, and in 2013 for both leaves grown at the UNAM pier meadow (ANOVA, P >0.05; Fig. 2b ). Unfortunately, no data are available for leaf #3 from 1995. Further analysis on the second youngest leaf of the shoot (leaf #2) on samples collected in 1995 found significantly higher CaCO 3 content for the back reef leaves relative to the content determined for leaves grown at the UNAM-Pier site (Student’s t -test, P <0.001). However, these differences were reversed in September 2013 (Student’s t -test, P <0.001; Fig. 2b ). Electron microscopy and X-ray microanalysis Electron microscopy (SEM, JSM-6390/LGS JEOL) and X-ray microanalysis (AXS. INCAx-ACT OXFORD system with X-ray detector free of liquid nitrogen, Oxford Instruments) were employed to find the CaCO 3 crystals on the seagrass blades. We analysed dry samples collected in the Puerto Morelos reef lagoon in 1995 and 2009 and in Tulum (Riviera Maya) in January 2013. Old leaves showed a dense coat on the surface formed by small crystals (2-3 μm long and 0.25 μm width) gathered within a matrix ( Fig. 3 ). This coat, which completely covered the leaf surface ( Fig. 3 ), had a weight composition of 21.6% Carbon, 42.4% Oxygen, 24.5% Calcium, 2.75% Magnesium, 2.9% Sodium and 5.78% Chloride, confirming the presence of CaCO 3 crystals within an organic matrix (atomic composition: 32.9% C; 48.5 O; 11.2% Ca; 2% Mg; 2.3% Na; and 2.98% Cl; see Supplementary Fig. 1a ). The shape and size of the carbonate crystals match the aragonite needles collected in whitings and bottom sediments of the Bahama Bank [17] , [18] ( Fig. 4 ). Crystals showed poorly developed faces with pointed terminations, as indicated by Gischler et al. [10] ( Figs 3 and 4c,d ). Semi-burned leaves, however, showed crystals with four well-developed faces ( Fig. 4a,b ). Further analysis concerning the type of crystal precipitated was achieved through the use of Feigl’s solution [48] , which stains aragonite crystals black leaving calcite crystals unstained [48] . Feigl’s solution confirmed that aragonite is the CaCO 3 crystallization form of the needles precipitated by T. testudinum ( Supplementary Fig. 2 ). Aragonite crystals were also found inside the leaf ( Figs 3c and 5 ). X-ray microanalysis allowed identification of crystals in an organized position inside the cell walls ( Fig. 6 , and Supplementary Fig. 1b ). The CaCO 3 deposits of the epidermal cell walls showed much lower organic carbon content than the external carbonate coat (cell wall atomic composition: 14.4% C; 55% O; 26.6% Ca; 3.6% Mg; see Supplementary Fig. 1b ; and CaCO 3 atomic composition: 12% C; 48% O; 40% Ca). This external coating was not observed in the young leaf segments, allowing visualization of the characteristic fenestrated cuticle of the seagrass leaf ( Fig. 7 ). A progressive change in the shape of the leaf cuticle was observed from a sunken wall surrounding each epidermal cell in the youngest fragments ( Figs 7a,b and 8a ), towards a convex wall ( Fig. 7c ). This change in the cuticle shape could result from the internal accumulation of aragonite crystals within the epidermal cell walls. We observed abundant crystals in the internal side of the leaf cuticle in samples that still did not show the external CaCO 3 coat ( Fig. 8e,f ). X-ray microanalysis allowed identification of CaCO 3 in small cuticle exudates on young leaf fragments (see Fig. 8a,b ; and Supplementary Fig. 1c ) despite aragonite needles being apparently absent (atomic composition: 33.6% C; 43.3 O; 16.8% Ca; 0.8% Mg; 2.1% Na; and 3.4% Cl see Supplementary Fig. 1c ). Clusters of needles were also observed on older fragments, coming out through the cuticle hole ( Fig. 7f ) and progressively extending on the blade in an organized structure ( Figs 3a , 7e ), until forming a dense external coating in the oldest fragments and leaves ( Figs 5a,g and 8c,d ). 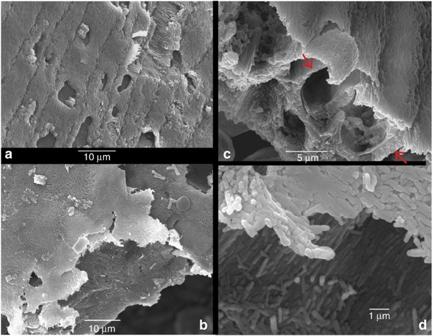Figure 3: SEM images of the external carbonate deposits. Multiple views of CaCO3deposits precipitated on leaf blades ofThalassia testudinumcollected in 1995. (a) Deposits precipitated in an organized shape along epidermal cells. (b) Detail of the different layers of the CaCO3deposits peeling off from the leaf surface. (c) Close-up of the epidermal cell layer showing the CaCO3deposits above the cuticle and around the cells. Arrows indicate the position of the internal deposits. (d) Close-up of the aragonite crystals within the external carbonate coat. Figure 3: SEM images of the external carbonate deposits. Multiple views of CaCO 3 deposits precipitated on leaf blades of Thalassia testudinum collected in 1995. ( a ) Deposits precipitated in an organized shape along epidermal cells. ( b ) Detail of the different layers of the CaCO 3 deposits peeling off from the leaf surface. ( c ) Close-up of the epidermal cell layer showing the CaCO 3 deposits above the cuticle and around the cells. Arrows indicate the position of the internal deposits. ( d ) Close-up of the aragonite crystals within the external carbonate coat. 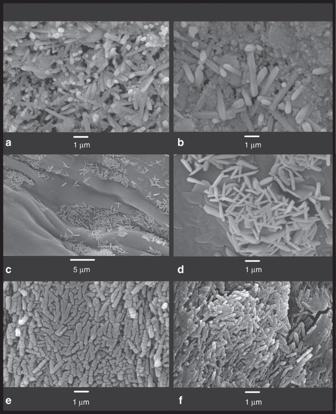Figure 4: SEM images of the seagrass crystals. SEM images of the seagrass aragonite crystals showing similar size and shape with the sedimentary non-skeletal needles18,19: (a,b) internal crystals within semi-burned leaves; (c,d) view of young CaCO3deposits on basal leaf fragments of the second youngest leaf; and (e,f) view of the CaCO3deposits on old leaves. The first two images (a,b) correspond to leaves collected in the reef lagoon of Puerto Morelos in April 2013. The four other images (c–f) correspond to leaves collected in Tulum (Riviera Maya, Mexico) in January 2013. Full size image Figure 4: SEM images of the seagrass crystals. SEM images of the seagrass aragonite crystals showing similar size and shape with the sedimentary non-skeletal needles [18] , [19] : ( a , b ) internal crystals within semi-burned leaves; ( c , d ) view of young CaCO 3 deposits on basal leaf fragments of the second youngest leaf; and ( e , f ) view of the CaCO 3 deposits on old leaves. The first two images ( a , b ) correspond to leaves collected in the reef lagoon of Puerto Morelos in April 2013. The four other images ( c – f ) correspond to leaves collected in Tulum (Riviera Maya, Mexico) in January 2013. 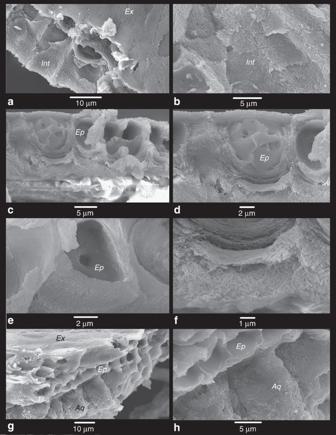Figure 5: SEM images of the internal and external seagrass carbonate deposits. SEM images of the seagrass CaCO3deposits: (a) Paradermal-horizontal view of the external (Ext) and internal (Int) sides of the leaf cuticle; (b) close-up of the internal side; (c,d) transversal-vertical views of the leaf showing the single epidermal layer (Ep) and the CaCO3deposits between the cells; (e,f) close-ups of the epidermal cell wall showing the abundant presence of aragonite crystals; and (g,h) view of the CaCO3deposits on the aerenquima cell walls (Aq). Full size image Figure 5: SEM images of the internal and external seagrass carbonate deposits. SEM images of the seagrass CaCO 3 deposits: ( a ) Paradermal-horizontal view of the external ( Ext ) and internal ( Int ) sides of the leaf cuticle; ( b ) close-up of the internal side; ( c , d ) transversal-vertical views of the leaf showing the single epidermal layer ( Ep ) and the CaCO 3 deposits between the cells; ( e , f ) close-ups of the epidermal cell wall showing the abundant presence of aragonite crystals; and ( g , h ) view of the CaCO 3 deposits on the aerenquima cell walls ( Aq ). 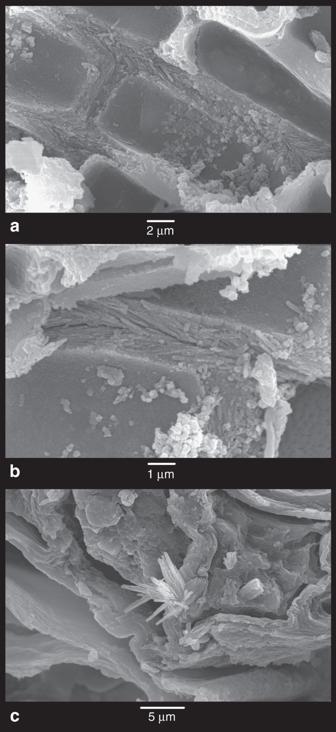Figure 6: SEM images of internal cell-wall carbonate deposits. SEM images of internal seagrass CaCO3deposits: (a,b) horizontal views from above of the cell wall of an epidermal cell showing the organized position of the crystals inside the wall (atomic composition: 33.5% C; 43.3% O; 16.9% Ca; 0.8% Mg; 2.1% Na; and 3.4% Cl); (c) transversal view of an epidermal cell showing the needles coming out from the wall. This cell also shows a large calcium oxalate crystal inside the cytoplasm, as described by Dobbset al.60 Full size image Figure 6: SEM images of internal cell-wall carbonate deposits. SEM images of internal seagrass CaCO 3 deposits: ( a , b ) horizontal views from above of the cell wall of an epidermal cell showing the organized position of the crystals inside the wall (atomic composition: 33.5% C; 43.3% O; 16.9% Ca; 0.8% Mg; 2.1% Na; and 3.4% Cl); ( c ) transversal view of an epidermal cell showing the needles coming out from the wall. This cell also shows a large calcium oxalate crystal inside the cytoplasm, as described by Dobbs et al. 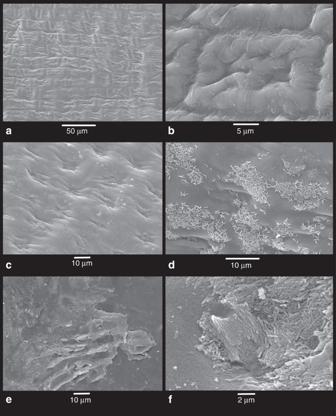Figure 7: Changes in the cuticle shape and development of the external aragonite deposits. SEM views of the progressive development of external CaCO3deposits onThalassia testudinumleaves. (a–c) Images of young leaf fragments showing a cuticle free of CaCO3crystals, where the fenestrate morphology of the seagrass cuticle and a progressive change in the cuticle shape from a concave-sunken wall surrounding the epidermal cell (a,b) towards a convex-filled wall (c) is visibly evident. (d–f) More mature leaf fragments showing an increasing presence of crystals, where (d,e) a progressive development of the carbonate coating and (f) close-up of a cluster of needles coming out through a cuticle hole, are visible. [60] Full size image Figure 7: Changes in the cuticle shape and development of the external aragonite deposits. SEM views of the progressive development of external CaCO 3 deposits on Thalassia testudinum leaves. ( a – c ) Images of young leaf fragments showing a cuticle free of CaCO 3 crystals, where the fenestrate morphology of the seagrass cuticle and a progressive change in the cuticle shape from a concave-sunken wall surrounding the epidermal cell ( a , b ) towards a convex-filled wall ( c ) is visibly evident. ( d – f ) More mature leaf fragments showing an increasing presence of crystals, where ( d , e ) a progressive development of the carbonate coating and ( f ) close-up of a cluster of needles coming out through a cuticle hole, are visible. 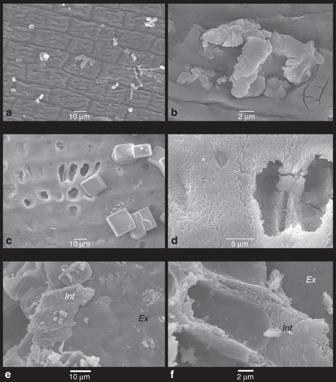Figure 8: Variation in the external presence of crystals. SEM views of the external surface ofThalassia testudinumleaves. Images of young leaf fragments (a,b), old fragments (c,d) and intermediate steps between them (e,f). (a) View of the fenestrated morphology of the seagrass cuticle and its sunken shape around each epidermal cell; (b) close-up of a small CaCO3deposit emerging from the cuticle (see microanalysis inSupplementary Fig. 1cconfirming the presence of CaCO3); (c) general view of a dense CaCO3deposit formed on an old leaf fragment; (d) close-up of this deposit allowing imaging of aragonite needles and its thickness (leaf cuticle is hardly seen deep into the holes). (e,f) Images of intermediate leaf fragments showing minimal presence of crystals on the external surface, but significant presence in the internal side (the images show the seagrass leaf cuticle turned up at the edge and placing the internal side(Int)on the top of the external side(Ex). Full size image Figure 8: Variation in the external presence of crystals. SEM views of the external surface of Thalassia testudinum leaves. Images of young leaf fragments ( a , b ), old fragments ( c , d ) and intermediate steps between them ( e , f ). ( a ) View of the fenestrated morphology of the seagrass cuticle and its sunken shape around each epidermal cell; ( b ) close-up of a small CaCO 3 deposit emerging from the cuticle (see microanalysis in Supplementary Fig. 1c confirming the presence of CaCO 3 ); ( c ) general view of a dense CaCO 3 deposit formed on an old leaf fragment; ( d ) close-up of this deposit allowing imaging of aragonite needles and its thickness (leaf cuticle is hardly seen deep into the holes). ( e , f ) Images of intermediate leaf fragments showing minimal presence of crystals on the external surface, but significant presence in the internal side (the images show the seagrass leaf cuticle turned up at the edge and placing the internal side (Int) on the top of the external side (Ex ). Full size image An increasing presence of epibionts was also observed on the external surface of the seagrass blade (see Supplementary Fig. 3 ). Diatoms were only visible on the youngest segments, free of the CaCO 3 coat, as previously reported [14] . However, our observations differ from previous descriptions [14] , as no overlapping of epibiont layers was found. Moreover, the carbonate deposits observed on the blade by these authors [14] were interpreted as coralline incrusting algae, but they are similar to the seagrass coating described in this study and strongly differ from coralline algal deposits. Coralline-encrusting algae have a well-defined shape and are formed by smaller calcite crystals, nanograins (<1 μm) as the main components (see Supplementary Fig. 3e,f ). According to our re-interpretation of previous images [14] as well as the findings shown in the current study, we propose that the progression of the external deposits on the seagrass blade may stop diatom colonization favouring the growth of other epibionts such as coralline-encrusting algae. These algae, which have a carbonate crystallization form of high-magnesium calcite, are the main component of the epibiont community of T. testudinum leaves in the coral reef habitat [14] . The current study provides multiple lines of evidence that support the conclusion that T. testudinum can be a biological source for the lime mud sediments produced in reefs and carbonate platforms along the Caribbean and Gulf of Mexico. While coralline-encrusting algae and diatoms are both important components of the epibiont community of T. testudinum leaves, our results explain the abundance of nanograin crystals [10] , [14] and coccoliths [10] in the finest mud fraction (<4 μm) of sediments from areas where T. testudinum is the dominant seagrass. Sediments from southern Belize and Bahía Almirante, Panama are particularly enriched in nanograins and high-magnesium calcite precipitates [49] . Our study, however, does not explain the biological mechanism behind seagrass calcification. We documented large seasonal and spatial variation that still needs to be understood. Basic information on the biological process and its regulation are needed before seagrass carbonate production can be incorporated into any carbon budget. Moreover, we still need to elucidate the magnitude of seagrass contribution to the carbonate factory through quantification of the direct gross carbonate production and the magnitude of carbonate losses due to dissolution and/or removal by oceanographic circulation flows. The strong circulation pattern of the Puerto Morelos reef-lagoon results in a very short water residence time (3 h) under normal wave conditions, with rapid expulsion of the continuous wave-induced water flow entering above the reef crest [50] . The fast circulation flowing through northern and southern channels [50] may explain the lack of local accumulation of lime mud in the sediment. Similar reductions in the finest mud fraction of the sediment (<4 μm) have been documented for northern Belize [10] . Therefore, the direct contribution of T. testudinum to local carbonate mud production will depend on the balance between carbonate production and dissolution [29] and the capacity of the environment to retain the small crystals. Other processes related to the decomposition rates of seagrass leaf debris and the migration of the carbonate mud associated with regional and/or local marine currents, tides and/or storms will help to elucidate the relative importance of the seagrass contribution to the accretion rates of tropical banks. Coral reef primary producers together with coccolithophorids in the open ocean are responsible for more than half of the world’s CaCO 3 production [51] . Coral reefs only account for 0.02% of the open ocean area, but their productivity is 200 times higher than that of coccolithophorids [52] . Therefore, coral reefs together with other neritic environments such as tropical banks, Halimeda bioherms, tropical-temperate shelves and boreal-polar shelves, which all occupy much smaller areas than the open ocean, are considered to produce as much carbonate as the open ocean [52] . T. testudinum is the builder of a key marine habitat in the coral reef system along the Caribbean and Gulf of Mexico. This ecosystem engineer has the capacity to retain significant amounts of organic blue-carbon through clonal growth, providing the habitat for important reef calcifiers (that is, codiacean algae and leaf epibionts). While seagrass biomass is known for stabilizing large volume of sediments, through the production of aragonite needles documented in the current study, T. testudinum beds could act as sources of inorganic carbon in the form of carbonate lime mud for the tropical carbonate factory. Thus, collectively, the evidence presented here indicates that turtlegrass may have a more important contribution to the capacity of the ocean to retain carbon than has thus far been considered. However, further research is required to fully understand the capacity of seagrass beds to significantly contribute to the accretion rate of tropical banks. Future research will also clarify whether seagrass calcification is a general phenomenon or is exclusive to this tropical species. This information is key for the evaluation of the contribution of seagrass calcification to the oceanic carbon cycle and the analysis of current and future impacts of ocean acidification, global warming and/or other local factors on oceanic lime mud production. Determination of seagrass calcification rates Calcification rates were determined using the alkalinity anomaly principle based on the ratio of two equivalents of total alkalinity per mole of CaCO 3 precipitated [31] . For alkalinity measurements, we used a modified spectrophotometer procedure as described by Yao & Byrne [53] and used in Colombo-Pallota et al. [54] for coral calcification determinations. Triplicate analyses for each sample were performed giving a s.d. for alkalinity measurements of less than 5 μmol l −1 . Microtitration with 0.3 N HCl was carried out at a rate of 8 μl min −1 using a glass syringe (Hamilton Company, Reno, USA) fitted to a syringe pump (Kd Scientific Inc., Holliston, USA) into a 1-cm length cuvette. Bromocresol Green (BCG; Sigma Aldrich, Steinheim, Germany) was added to the water sample before the microtritration and after gently bubbling the sample with N 2 for at least 10 min. During the microtritration, changes in the absorbance at 444, 616 and 750 nm were continuously recorded with an Ocean Optics USB4000 spectrophotometer (Ocean Optics, Dunedin, USA) and using a xenon light source (PX-2, Ocean Optics, Dunedin, USA). Water temperature was recorded at the end of the microtritration with a digital thermometer. For the accurate assessment of this determination, we used certified reference material (known total alkalinity) from the Marine Physical Laboratory (Scripps Institution of Oceanography, USA). The incubations were performed with freshly collected and filtered (0.45 μm) oceanic water collected directly from the Yucatan Current [55] outside from the reef lagoon of Puerto Morelos. The oceanic water is extremely poor in nutrient content [56] , and thus cannot induce other leaf uptake processes that could be misinterpreted as calcification. For these determinations, we used 2-cm long fragments (1.5–2 cm 2 ) of the second youngest leaf of the shoot, free of epibionts, selected between 3 and 6 cm of distance from the basal meristem. The second youngest leaf of T. testudinum is less affected by epibiont growth and damage accumulation, and mature enough to show the physiological response. We used incubation times of 45 min in 12 ml water-jacked chambers (DW3, Hansatech Instruments Ltd., Norfolk, UK) under saturating light (500 μmol quanta m −2 s −1 ) to perform simultaneous determinations of maximum photosynthetic ( P max ) and calcification ( G max ) rates. After the light incubation, water was collected for the calcification rate determinations. Incubation time was chosen from previous tests, as it showed the higher rates and lower variation among replicates. We found for net P max rates of 2.5±0.3 μmol O 2 cm −2 h −1 at 28.5 °C, a ΔpH of 0.16±0.04 and DIC losses of 182.9±4.3 μmol l −1 ( n =4). The induced alkalinity changes ranged between 100 and 200 μmol l −1 . Leaf respiration was determined after light incubations, maintaining leaf fragments in darkness for another 10–15 min. The leaves of T. testudinum have the ability to use β-carboxylation as a carbon concentration mechanism (CCM) [57] , which enhances the internal CO 2 concentration at Rubisco, the primary site of carbon fixation, through the production of C4 molecules as malate, oxalate and aspartate. β-Carboxylation maintains seagrass photosynthetic activity without a continuous external DIC supply. We found that 33% of the total carbon losses (DIC) through photosynthesis and calcification need to be supported by the seagrass metabolism. This observation implies that estimates of the impact of seagrass photosynthesis and calcification on the habitat carbon budget need to consider the internal seagrass carbon supply. Seagrass metabolic rates were measured polarographically using Clark-type O 2 electrodes. A circulating bath with a controlled temperature system (RTE-100/RTE 101LP; Neslab Instruments, Postsmouth, NH, USA) allowed maintenance of the selected temperature during the incubations. Light was provided by a LS2-high intensity tungsten-halogen light source (Hansatech Instruments, Norfolk, UK). The leaves of T. testudinum are characterized by small dark respiration rates [58] , [59] . The low metabolic activity under dark conditions allows for recognition of potential bacterial contamination during the incubations, as large variation among replicates reflects the occurrence of respiratory activity not related to the seagrass leaf respiration. No such contamination was observed in any dark respiration determination. Leaf segments treated with DCMU (3′-(3,4-dichlorophenyl)-1′1′-dimethyl urea) as shown in Enríquez et al. [58] were incubated at 28 °C for 45 min under 500 μmol quanta m −2 s −1 . The herbicide DCMU is a known inhibitor of the photosynthetic electron flow beyond Qa. Acetazolamide (AZ), an inhibitor of the external carbonic anhydrase activity, was dissolved in DMSO to a final concentration of 0.6 mM. Leaf segments treated with AZ were incubated for 30 min under 28 °C and 500 μmol quanta m −2 s −1 . Seasonal monitoring Plants were collected at 2.5 m depth in the back reef meadow (site 5 in Enríquez & Pantoja-Reyes [39] ). Leaf segments between 4 and 6 cm from the leaf meristem were incubated for 30 min in 12 ml water-jacked chambers (DW3, Hansatech Instruments, Norfolk, UK) under a saturating light intensity of 500 μmol quanta m −2 s −1 . Between 9 and 10 leaf segments were characterized in each determination. Instantaneous metabolic rates were measured at the same temperature as recorded in situ at sampling, using a circulating bath with a controlled temperature system (RTE-100/RTE 101LP; Neslab Instruments, Portsmouth, NH, USA). Oxygen evolution measurements were performed using Clark-type O 2 electrodes (Hansatech) calibrated with air- and N 2 -saturated filtered seawater. Photosynthetic rates under saturating light conditions ( P max ) were determined at 500 μmol quanta m −2 s −1 , and leaf respiration was determined under 10–15 min in darkness. Dates of sampling were as follows: 18 March 2003; 15 April 2003; 2 May 2009; 11 June 2009; 26 June 2003; 20 July 2003; 7 August 2009; 18 August 2009; 26 November 2009; 4 December 2009. Temperature and water motion data from 2009 were measured in the middle of the reef lagoon, right in front of the UNAM pier at 3.3 m depth, by the Oceanographic and Meteorological Academic Service (SAMMO) of the UNAM in Puerto Morelos. Variation in water motion (m s −1 ) was registered with an Acoustic Doppler Velocimeter (Argonaut-ADV, SonTek/YSI). Measurements were recorded at 2 cm from the sediment, using a 6 mm diameter × 9 mm high cylinder. Estimations of seagrass carbonate budgets For calculations of the daily and annual carbonate production, it was assumed 10 h per day under maximum photosynthesis ( P max ), as previous work has documented for this lagoon that T. testudinum leaves are exposed to supersaturating light levels for most of the day [58] , and 14 h under dark calcification rates assuming dark calcification as half of the rate determined at P max . We did not consider potential enhancement of carbonate production under subsaturating photosynthesis. We calculated gross carbonate production assuming 153 days of positive calcification (5 months) per year and using the average rate determined for 2009, and using the average between two consecutive determinations and calculating the carbonate production for this period. The annual gross carbonate production was estimated by adding the carbonate production calculated for each period ( Table 1 ). These values do not consider carbonate dissolution and do not consider all the seasonal variability exhibited by carbonate lime mud production in the reef lagoon of Puerto Morelos during 2009. They provide an estimation of the magnitude of gross seagrass carbonate production for this Caribbean reef lagoon. Loss on ignition analysis The leaf segments analysed were free of macroscopic epibionts and corresponded to the second youngest growing leaf of the shoot (leaf #2) for the samples collected in 1995. In 2013, we analysed leaf number 2 and leaf number 3 (the oldest leaf of the shoot) separately. For this quantification, we compared leaves grown in two seagrass meadows: close to the back reef and adjacent to the UNAM pier. Shoots growing at the UNAM pier were larger in length than in the back reef (see description by Enríquez and Pantoja-Reyes [39] ). For the back reef meadow, we also compared 1995 leaves, which strongly differed in size, from shoots located in the centre of the meadow (short leaves) or adjacent to massive coral colonies (large leaves). Such differences were less apparent in 2013. Samples collected in May 1995 were analysed in the Freshwater Biological laboratory, Denmark, a month after sampling. Samples collected in 2013 were analysed immediately after sampling at the UNAM facilities in Puerto Morelos (Mexico). How to cite this article: Enríquez, S. et al. Direct contribution of the seagrass Thalassia testudinum to lime mud production. Nat. Commun. 5:3835 doi: 10.1038/ncomms4835 (2014).